Structure-guided evolution of cyan fluorescent proteins towards a quantum yield of 93% Cyan variants of green fluorescent protein are widely used as donors in Förster resonance energy transfer experiments. The popular, but modestly bright, Enhanced Cyan Fluorescent Protein (ECFP) was sequentially improved into the brighter variants Super Cyan Fluorescent Protein 3A (SCFP3A) and mTurquoise, the latter exhibiting a high-fluorescence quantum yield and a long mono-exponential fluorescence lifetime. Here we combine X-ray crystallography and excited-state calculations to rationalize these stepwise improvements. The enhancement originates from stabilization of the seventh β-strand and the strengthening of the sole chromophore-stabilizing hydrogen bond. The structural analysis highlighted one suboptimal internal residue, which was subjected to saturation mutagenesis combined with fluorescence lifetime-based screening. This resulted in mTurquoise2, a brighter variant with faster maturation, high photostability, longer mono-exponential lifetime and the highest quantum yield measured for a monomeric fluorescent protein. Together, these properties make mTurquoise2 the preferable cyan variant of green fluorescent protein for long-term imaging and as donor for Förster resonance energy transfer to a yellow fluorescent protein. After the cloning of green fluorescent protein from Aequorea victoria , colour variants were created by mutagenesis [1] . The mutation of the central residue of the chromophore from a tyrosine to a tryptophan resulted in a blueshift of the absorption peak, but strongly reduced the fluorescence [2] . A few rounds of mutagenesis in the chromophore cavity were necessary to accommodate the increased bulk of tryptophan and restore an acceptable level of fluorescence in Enhanced Cyan Fluorescent Protein (ECFP) (quantum yield (QY)=0.36) [3] . Subsequently, cyan fluorescent proteins have been widely applied as donors in Förster resonance energy transfer (FRET) experiments in combination with a yellow fluorescent protein (YFP) as acceptor [4] , [5] . Structural analysis of ECFP revealed that the mutations resulted in alternate conformations of the seventh strand of the β-barrel [6] , [7] . Rational design based on these alternate conformations led to an improved variant called Cerulean (QY=0.49), containing the two mutations Y145A and H148D [8] . Nevertheless, Cerulean still exhibited structural heterogeneity of the seventh strand [7] . A different study, employing site-directed mutagenesis to evaluate the effect of individual mutations, led to the development of Super Cyan Fluorescent Protein 3A (SCFP3A) (QY=0.56), which harbours only the H148D mutation [9] . Apart from moderate brightness, all these mutants suffer from complex fluorescence decay kinetics, complicating the analysis of lifetime-based FRET measurements. Recently, a family of much improved variants were identified by a combination of site-directed mutagenesis and a new fluorescence lifetime-based screening [10] . Surprisingly, it took only a single mutation of a residue that is part of the chromophore, T65S, to significantly improve the brightness of SCFP3A. The resulting variant, mTurquoise, is 50% brighter owing to its high QY of 0.84 and exhibits a mono-exponential fluorescence decay [11] . Another mutant, mTurquoise-148G/224L (mTurquoise-GL), exhibits one of the longest fluorescence lifetimes observed for any fluorescent protein. The residues of ECFP, which have been mutated to successively yield Cerulean, SCFP3A, mTurquoise and mTurquoise-GL, are highlighted in yellow in Fig. 1 and listed in Supplementary Table S1 . Recently, improved CFP variants based on Cerulean were described [12] . mCerulean2 was obtained from Cerulean using several mutations, which include the critical H148G mutation, previously identified in mTurquoise-GL. Subsequently, mCerulean3 was considerably improved by the single mutation T65S, which is also responsible for the high QY of mTurquoise. The QYs were significantly improved to 0.60 and 0.87 for mCerulean2 and mCerulean3, respectively. 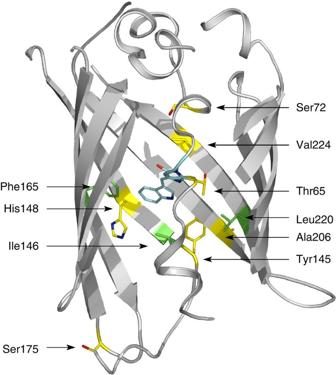Figure 1: ECFP residues examined in this work. The secondary structure of ECFP is drawn in light grey, and the chromophore in cyan. Residues that have been mutated in the previously described improved variants are shown in yellow, and those mutated in the present work in green. Figure 1: ECFP residues examined in this work. The secondary structure of ECFP is drawn in light grey, and the chromophore in cyan. Residues that have been mutated in the previously described improved variants are shown in yellow, and those mutated in the present work in green. Full size image Here we first present the high-resolution X-ray structures of SCFP3A and mTurquoise, whose examination explains the progressive improvement in fluorescence QY and fluorescence lifetime. Our structural analysis unveiled one suboptimal residue, Ile146, which was targeted for further improvement. Using our fluorescence lifetime-based screening method, we then identified the I146F mutation that confers a higher lifetime. The X-ray structure of this mutant, dubbed mTurquoise2, reveals that the mutated residue contributes to an improved packing of the chromophore through many further van der Waals (vdW) interactions. This increases the QY to 0.93, which is now the highest for a monomeric fluorescent protein. Thorough in vivo characterization of mTurquoise2 shows an almost 20% gain in brightness in mammalian cells, high photostability and improved performance as a donor for FRET to a YFP. The seventh strand adopts one single conformation in SCFP3A Previously, we have reported the SCFP3A variant with a threonine at position 65, which displayed improved brightness over ECFP [9] . To examine the underlying mechanism for the improvement, the structure of SCFP3A was determined. The X-ray structure of SCFP3A was solved at 1.59 Å resolution in the same experimental conditions as ECFP, which made a close comparison between these structures possible. The root mean square deviation (r.m.s.d.) plot on main-chain C α atoms between SCFP3A and ECFP shows that both structures are very similar (r.m.s.d. of 0.21 Å on all C α 's), except for the seventh strand, the adjacent loop [131–143] and two other loops ( Supplementary Fig. S1 ). In particular, the S175G mutation explains the significant difference on the loop connecting the eighth and ninth strands. The most striking feature of the structure of SCFP3A is that the whole main chain of its seventh strand is in a single conformation as demonstrated by the continuous electron density on the main chain of residues 144 and 145, unlike the structures of ECFP and Cerulean ( Fig. 2a ). Analysis of the hydrogen-bond (H-bond) pattern between adjacent β-strands shows that the seventh and tenth strands are perfectly locked in SCFP3A up to residues 144 and 207, whereas the last H-bond of these strands is present in only one conformation of ECFP, but in none of the Cerulean conformations ( Fig. 2b ). 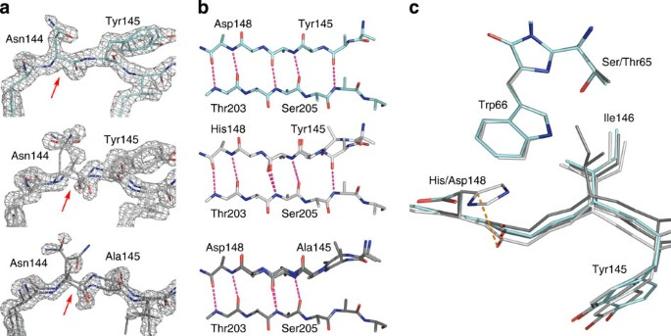Figure 2: Structural characterization of SCFP3A. (a) Comparison of the electron density of the seventh strand in various CFP mutants. The 2Fo–Fc map is superimposed on residues 143–146 and contoured at a 1.6σlevel for SCFP3A (light blue), ECFP (light grey) and Cerulean (dark grey). Red arrows indicate the position of the Cα–C bond in Asn144, on which the electron density is discontinuous in ECFP and Cerulean, and continuous in SCFP3A. As a consequence, the structures of ECFP and Cerulean had to be modelled with two conformations of the main chain of the seventh strand, whereas SCFP3A could be modelled with one single conformation. (b) H-bond pattern bridging the seventh and tenth strands in SCFP3A, ECFP and Cerulean (from top to bottom). The alternate conformation of the seventh strand is shown in white. (c) Positions of residues 145, 146 and 148 on the seventh strand relative to the chromophore in ECFP, Cerulean and SCFP3A. Figure 2: Structural characterization of SCFP3A. ( a ) Comparison of the electron density of the seventh strand in various CFP mutants. The 2 F o– F c map is superimposed on residues 143–146 and contoured at a 1.6 σ level for SCFP3A (light blue), ECFP (light grey) and Cerulean (dark grey). Red arrows indicate the position of the C α –C bond in Asn144, on which the electron density is discontinuous in ECFP and Cerulean, and continuous in SCFP3A. As a consequence, the structures of ECFP and Cerulean had to be modelled with two conformations of the main chain of the seventh strand, whereas SCFP3A could be modelled with one single conformation. ( b ) H-bond pattern bridging the seventh and tenth strands in SCFP3A, ECFP and Cerulean (from top to bottom). The alternate conformation of the seventh strand is shown in white. ( c ) Positions of residues 145, 146 and 148 on the seventh strand relative to the chromophore in ECFP, Cerulean and SCFP3A. Full size image The single conformation of the seventh strand in SCFP3A can be explained by the single mutation H148D. Just like in Cerulean, the side chain of residue 148 is rotated away from its conformation in ECFP, in which it is parallel to the surface of the protein, oriented towards the bulk solvent ( Fig. 2c ). As a consequence, there is significantly more room for the carbonyl group of Ser147, which moves by 0.4 Å towards the chromophore. This change propagates further down the strand, resulting in successive rearrangements that allow for the stabilization of the main chain of residues [143–146], which corresponds to the conformation closer to the chromophore in ECFP. Locking down the seventh strand in one conformation provides a sound explanation for the fluorescence QY improvement in SCFP3A compared with ECFP. In ECFP, it has been shown that the strand undergoes a dynamical equilibrium on the nanosecond timescale between at least two conformations, which eventually brings Ile146 in collision conditions with the chromophore, causing fluorescence quenching [7] . In SCFP3A, as there is only one conformation of the strand, there cannot be a comparably large-amplitude dynamical equilibrium of the main chain, and movements of the Ile146 side chain are restricted compared with the ECFP situation, reducing the likelihood of fluorescence quenching. This improvement is of a nature different from that observed for Cerulean. In the latter mutant, the extra Y145A mutation replaces a bulky residue by a much smaller one, which allows the seventh strand to slide into the core of the protein ( Fig. 2c ), yet imperfectly, as two conformations of the main chain are still observed [7] . One of these conformations allows Ile146 to be packed onto the chromophore in a stabilizing manner. In the other conformation, Ile146 is still positioned on a flexible strand and, therefore, a collisional quenching mechanism by its side chain still exists. In other words, the H148D mutation in Cerulean helped to cure partly the defects of ECFP, but the Y145A mutation introduced a new one. The single conformation of the seventh strand explains why SCFP3A is brighter than ECFP and Cerulean [10] . The chromophore-stabilizing H-bond is stronger in mTurquoise The CFP variant mTurquoise has a single point mutation T65S relative to SCFP3A, which increases both fluorescence lifetime and QY substantially [10] . To examine the reason for the improved properties, we determined the 1.47-Å resolution crystal structure of mTurquoise, which turned out to be extremely close to that of SCFP3A, at least for the positioning of C α atoms ( Supplementary Fig. S1 ; r.m.s.d. of 0.10 Å). This was unsurprising, because the difference in amino-acid sequence was small (one less methyl group in Thr65), and at the same time puzzling, because the large improvement in brightness called for significant structural changes. To ensure that our mTurquoise crystals contain the physiologically relevant state of the protein, ultraviolet-visible light absorption and fluorescence emission spectra, as well as time-correlated single photon counting (TCSPC) histograms, were recorded on crystals and compared with those of solution samples ( Fig. 3a ). Essential features, such as the position of the two peaks in absorption and fluorescence spectra and the single, long fluorescence lifetime, are conserved. To unambiguously visualize the subtle differences between the two structures, we chose to calculate Fourier difference maps [13] , which is only possible when the crystals are reasonably isomorphous. This method has low model bias, as it is based on two sets of experimental structure factors and only one model of one protein (to provide calculated phases). 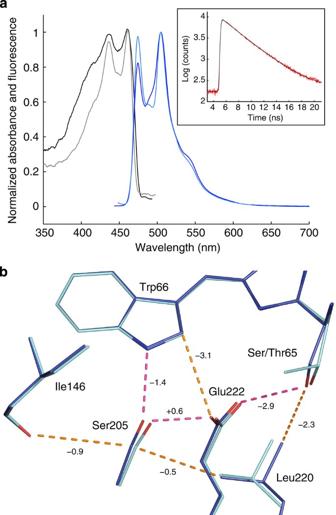Figure 3: Structural characterization of mTurquoise. (a) Ultraviolet–visible light absorption (black) and fluorescence emission (blue) spectra of mTurquoise in solution (light colours) and in the crystalline state (dark colours) at 100 K. Inset: TCSPC histogram of a mTurquoise crystal recorded at room temperature, of which a fluorescence lifetime of 3.55 ns is calculated. (b) Superimposition of the models of SCFP3A (cyan) and mTurquoise (blue). Hydrogen bonds are drawn in magenta, and vdW contacts are indicated in orange. Interaction energy gains between SCFP3A and mTurquoise in the excited state are indicated in kJ mol−1on the corresponding H-bonds or vdW contacts. Figure 3: Structural characterization of mTurquoise. ( a ) Ultraviolet–visible light absorption (black) and fluorescence emission (blue) spectra of mTurquoise in solution (light colours) and in the crystalline state (dark colours) at 100 K. Inset: TCSPC histogram of a mTurquoise crystal recorded at room temperature, of which a fluorescence lifetime of 3.55 ns is calculated. ( b ) Superimposition of the models of SCFP3A (cyan) and mTurquoise (blue). Hydrogen bonds are drawn in magenta, and vdW contacts are indicated in orange. Interaction energy gains between SCFP3A and mTurquoise in the excited state are indicated in kJ mol −1 on the corresponding H-bonds or vdW contacts. Full size image The resulting difference map ( Supplementary Fig. S2 ) shows that the T65S mutation induces a perturbation that is subsequently communicated to neighbouring residues. Examination of the map at ±4.5 σ lists eight major peaks around the chromophore, whose interpretation is significant in understanding the mechanism underlying the fluorescence improvement. Three of them occur on Ser/Thr65, indicating the disappearance of one methyl group and the displacement of the hydroxyl group towards Glu222. A further three major peaks are found on Leu220, where the arrangement of negative and positive difference densities indicates a complex displacement of Leu220 in mTurquoise compared with SCFP3A (displacement and rotation towards Glu222 and the chromophore). Finally, a strong pair of negative and positive difference densities is observed on Ser205, indicating a translation towards the seventh strand in mTurquoise. Therefore, the effects of the T65S mutation can be summarized as follows: removing the methyl group of Thr65 releases a strain on the C α of residue 65, and leaves some space that can be occupied by Leu220. Leu220 thus moves closer to the chromophore, and, through vdW contact, displaces Glu222 towards the chromophore as well (movement of 0.1 and 0.2 Å of the terminal oxygens). Similarly, Leu220 displaces the side chain of Ser205 towards the seventh strand by 0.3 Å through vdW contact ( Fig. 3b ). Finally, Ser205 presses on the carbonyl group of Ile146 through vdW interaction, which maintains the strand at a distance from the chromophore. To validate this scenario, which includes rather small atom displacements, we calculated interaction energy terms between pair-wise residues in the vicinity of the chromophore in both proteins, in both ground and excited states, with two different excitation schemes (vertical excitation and excited-state relaxation) ( Fig. 3b ; Supplementary Tables S2–S4 ; Supplementary Note 1 ). The first effect of the T65S mutation is to leave room for the establishment of a vdW interaction between Ser65 and Leu220. As a consequence, the already very strong H-bond-mediated interaction between residue 65 and Glu222 is strengthened further. Furthermore, the increased vdW interaction between the Ile146 main chain and Ser205 participates in rigidifying the whole environment of the chromophore, and limits potential quenching by the Ile146 side chain. Finally, and most importantly, the only H-bond stabilizing the chromophore, between Ser205 and the indole ring of Trp66, is strengthened by −2 kJ mol −1 in the excited state. In brief, the chromophore is better packed in mTurquoise, which limits non-radiative decay of its excited state and thus favours fluorescence. Rational design of mTurquoise2 Our structural analysis of CFP variants highlighted the rigidity of most of the residues surrounding the chromophore, except for Ile146, which shows a high variability in position and conformation between all four variants ( Fig. 4a ). Thus, we performed site-directed saturation mutagenesis at position 146, transformed bacteria and analysed colonies, using a recently developed fluorescence lifetime-based screening method [10] . A significant number of colonies exhibited a drastic decrease in lifetime, which showed the importance of that specific residue. We picked colonies with a high lifetime (around 4 ns), moderate lifetime (below 3.5 ns) and low lifetime (below 3 ns) and verified their lifetime in a second round of fluorescence lifetime analysis ( Fig. 4b ). Close inspection of the lifetimes showed that the mutants with 146F have an increased lifetime relative to mTurquoise. We also found N, G and Q at position 146, yielding a lifetime between 3.0 and 3.2 ns, and R and S, yielding a lifetime of 2.8 ns. The 146N corresponds to the residue in wild-type green fluorescent protein (GFP) and shows that this substitution is detrimental for the CFP lifetime. We chose to characterize the properties of mTurquoise-146F, mTurquoise-146G and mTurquoise-146S in more detail. We also performed mutagenesis at position 220, because of the markedly different position of Leu220 in mTurquoise compared with SCFP3A. Also, position 165 was targeted as a negative control, since Phe165 is, like Ile146, a hydrophobic residue located on the same side of the indole ring, but to the other side of the symmetry axis. We only observed variants with similar or lower lifetime. The effect of mutating position 165 on lifetime was strong (similar to 146), whereas the effect of mutagenesis of residue 220 was relatively mild ( Supplementary Fig. S3 ). 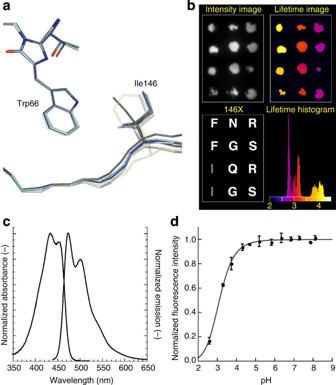Figure 4: Identification of mTurquoise2 and spectroscopic characterization. (a) Comparison of the Ile146 position in all known structures of CFP, highlighting its weak interaction with the chromophore (ECFP: light grey; Cerulean: dark grey; SCFP3A: light blue; mTurquoise: dark blue). The position of Phe146 in mTurquoise2 is shown as transparent green by anticipation. (b) Fluorescence lifetime imaging of bacterial colonies expressing 146X variants of mTurquoise with fluorescence intensities (upper left), and fluorescence modulation-based lifetimes (upper right). Sequencing revealed the identity of the residue at position 146 (lower left), with the corresponding residue in mTurquoise depicted in grey. Colonies with phenylalanine at 146 show an increased fluorescence lifetime, which can be discerned in the lifetime histogram as a separate peak around 4 ns, whereas the lifetime of mTurquoise is around 3.8 ns. The lifetime image is pseudo-coloured according to the scale shown in the histogram (values in ns). (c) Normalized absorption and fluorescence emission spectra of mTurquoise2. (d) pH dependence of mTurquoise2 fluorescence. Each point corresponds to the average of three measurements and is represented with the standard deviation. Data point interpolation (dark grey) results in a pKaof 3.1. Figure 4: Identification of mTurquoise2 and spectroscopic characterization. ( a ) Comparison of the Ile146 position in all known structures of CFP, highlighting its weak interaction with the chromophore (ECFP: light grey; Cerulean: dark grey; SCFP3A: light blue; mTurquoise: dark blue). The position of Phe146 in mTurquoise2 is shown as transparent green by anticipation. ( b ) Fluorescence lifetime imaging of bacterial colonies expressing 146X variants of mTurquoise with fluorescence intensities (upper left), and fluorescence modulation-based lifetimes (upper right). Sequencing revealed the identity of the residue at position 146 (lower left), with the corresponding residue in mTurquoise depicted in grey. Colonies with phenylalanine at 146 show an increased fluorescence lifetime, which can be discerned in the lifetime histogram as a separate peak around 4 ns, whereas the lifetime of mTurquoise is around 3.8 ns. The lifetime image is pseudo-coloured according to the scale shown in the histogram (values in ns). ( c ) Normalized absorption and fluorescence emission spectra of mTurquoise2. ( d ) pH dependence of mTurquoise2 fluorescence. Each point corresponds to the average of three measurements and is represented with the standard deviation. Data point interpolation (dark grey) results in a pK a of 3.1. Full size image The fluorescence lifetime of the I146F, I146G and I146S variants was measured in mammalian cells. The I146F mutant gave 3.8 and 4.0 ns for the phase and modulation lifetime, respectively, verifying the increased lifetime relative to mTurquoise ( Table 1 ). The lifetime values of 146G and 146S obtained from mammalian cells were similar to those observed in the lifetime screen (compare Table 1 and Fig. 4b ). The fluorescence lifetime-based screen for identifying variants with improved quantum yield [10] relies on the observation that the excited state lifetime of a fluorophore correlates with its fluorescence quantum yield. We then purified mTurquoise-146F and determined its quantum yield to be 0.93, which is an improvement of 10% over mTurquoise. Because of the improved lifetime and quantum yield, we dubbed the mTurquoise-146F variant mTurquoise2. During the characterization of mTurquoise2, another CFP variant with a high QY, mCerulean3, was published [12] . Therefore, we included mCerulean3 in the characterization. Table 1 Key properties of novel CFP variants. Full size table The extinction coefficient of mTurquoise2 was determined on purified protein and found to be 30,000 M −1 cm −1 , which is equal to mTurquoise and other CFP variants [7] , [9] , [10] , [14] . Extinction coefficients as high as 43,000 and 40,000 M −1 cm −1 were reported for Cerulean and mCerulean3, respectively [12] . However, these extinction coefficients were obtained using protein concentrations that were calculated based on a theoretical extinction coefficient of the protein instead of experimentally determined protein concentrations [15] . The values reported in this study are obtained using a protein determination assay on purified protein and by measuring the absorbance at 434 nm. It is of note that, as the assay is done with a bovine serum albumin standard, true protein concentrations may deviate by as much as 10% from the determined values. We observed that highly purified mTurquoise2 and mCerulean3 have almost identical absorption spectra ( Supplementary Fig. S4 ), with equal absorbances at 280 nm ( A 280 , representing the whole protein) as well as at 434 nm ( A 434 , representing the chromophore). Similar absorption spectra were previously obtained from purified SCFP3A ( Supplementary Fig. S4 ) and Cerulean [7] . These results again demonstrate that the extinction coefficients, which are proportional to A 434 / A 280 , are identical for all these cyan fluorescent proteins. To evaluate the brightness of mTurquoise2, the molecular brightness of single fluorescent proteins in solution was determined using fluorescence fluctuation spectroscopy (FFS). We observed a 10% increase in brightness relative to mTurquoise ( Table 1 ), which fits very well with the increase in quantum yield. Overall, the molecular brightness of the CFP variants correlates very well with their quantum yield, again arguing against differences in extinction coefficients between CFP variants. Spectroscopic characterization of mTurquoise2 revealed that absorption and fluorescence emission spectra are unaltered relative to its predecessor mTurquoise, representing bona fide CFP spectral characteristics ( Fig. 4c ). Notably, the higher quantum yield enhances FRET to YFPs. The calculated Förster radius for the mTurquoise2–mVenus [16] pair is 58.3 Å, which is 1 Å higher than that for mTurquoise–mVenus [10] . The fluorescence of mTurquoise2 is independent of pH over a large range and has a very low pK a of 3.1 ( Fig. 4d ). To examine the basis for the improved lifetime and QY of mTurquoise2, we solved the structure of mTurquoise2 at 1.31 Å resolution, which was found to be virtually identical to that of mTurquoise except for the position of the seventh strand. The most remarkable difference consists in the positioning of the bulky side chain of Phe146 that establishes a strong set of vdW interactions with the chromophore and the hydrophobic residues Ile167 and Val61 close by (compare Fig. 5a and b ). The interaction energy between residue 146 and the latter three residues in the excited state is increased by −12 kJ mol −1 between mTurquoise and mTurquoise2, and more than half of this gain is accounted for just by the Phe146–Trp66 interaction ( Supplementary Tables S3 and S4 ). As a consequence, the whole seventh strand is stabilized as shown by the decrease of relative crystallographic temperature factors ( B -factors), although the seventh strand is slightly pushed away towards the bulk solvent to accommodate for the increased size of the residue 146 side chain ( Fig. 4a ). The stabilization is remarkably illustrated by the fact that Tyr145 exhibits a single conformation of its side chain, unlike in SCFP3A and mTurquoise. Finally, the whole environment of the chromophore in the excited state is stabilized by −16 kJ mol −1 between mTurquoise and mTurquoise2 ( Supplementary Tables S3 and S4 ). This stabilization notably includes increased interactions of Glu222 with both Ser65 and Trp66 of the chromophore, and the formation of a vdW interaction between Ser205 and Phe146. Overall, our structural results evidence that the chromophore is stabilized from all sides, most importantly by the once dynamic seventh strand. 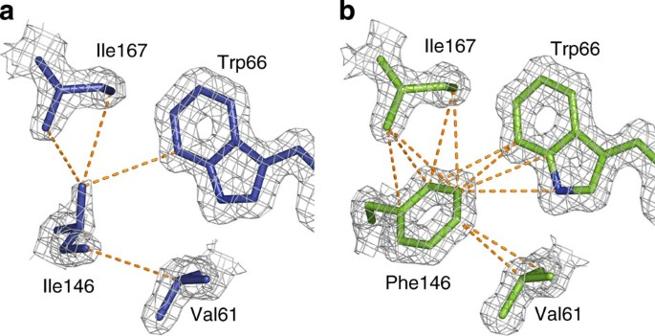Figure 5: Structural characterization of mTurquoise2. (a) Environment of residue 146 in mTurquoise and (b) in mTurquoise2. The electron density is represented on the mTurquoise (dark blue) and mTurquoise2 (green) models at a 1.6σlevel. Inter-atomic distances lower than 4.0 Å, characteristic of vdW interactions, are represented as dotted orange lines. The much greater number of such distances in mTurquoise2 illustrates the marked increase in stabilization of the chromophore by vdW interactions. Figure 5: Structural characterization of mTurquoise2. ( a ) Environment of residue 146 in mTurquoise and ( b ) in mTurquoise2. The electron density is represented on the mTurquoise (dark blue) and mTurquoise2 (green) models at a 1.6 σ level. Inter-atomic distances lower than 4.0 Å, characteristic of vdW interactions, are represented as dotted orange lines. The much greater number of such distances in mTurquoise2 illustrates the marked increase in stabilization of the chromophore by vdW interactions. Full size image Characterization of mTurquoise2 in vivo Previously, we established that mTurquoise has a mono-exponential lifetime by multifrequency fluorescence lifetime imaging microscopy (FLIM), which has been independently confirmed recently [11] . Multifrequency FLIM of mTurquoise2 in living mammalian cells demonstrated that it also has a mono-exponential fluorescence decay with a lifetime of 4.0 ns, which is an improvement of 0.2 ns relative to mTurquoise ( Supplementary Fig. S5 ). Next, the development of CFP fluorescence in growing Escherichia coli cultures was monitored to evaluate maturation speed. The observation that mTurquoise maturation is delayed by 1 h relative to SCFP3A and mCerulean [10] was reproduced ( Supplementary Fig. S6 ), but we noticed that mTurquoise2 maturation was almost as fast as SCFP3A, reversing the delay in maturation that was characteristic for mTurquoise. Subsequently, we measured the brightness in mammalian cells by quantitative co-expression of mTurquoise variants together with SYFP2 (mVenus-L68V) [9] , which is used as an internal control [10] . Using this assay, we found that the brightness of mCerulean3 is 95% relative to mTurquoise, and the brightness of mTurquoise2 is 118% relative to mTurquoise ( Table 1 , Supplementary Fig. S7 ). Considering the increase in QY of mTurquoise2 of 10%, the improved in vivo brightness is explained by increase in both quantum yield and maturation. Similar characterization of the I146G and I146S variants showed that the reduced lifetimes correlate with reduced quantum yields, as well as reduced in vitro and in vivo brightness ( Table 1 ). To evaluate its performance as a localization tag in living cells, mTurquoise2 was fused to a variety of proteins and localization signals. As shown in Fig. 6a–i , mTurquoise2 can be used to highlight cellular structures, including peroxisomes, actin filaments, nucleus, cytoplasm, plasma membrane, endoplasmic reticulum, microtubules and mitochondria. 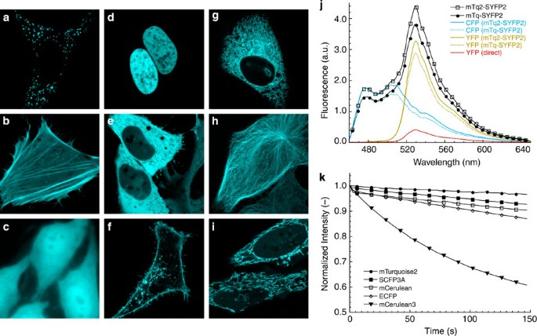Figure 6: Characterization of thein vivoproperties of mTurquoise2. (a–i) Fluorescence microscopy images of HeLa cells expressing mTurquoise2 fused to various proteins and targeting sequences (a peroxisomal targeting sequence, Lifeact, no fusion, histone 2A, a nuclear export sequence, a palmitoylation sequence, an endoplasmic reticulum targeting sequence, alpha-tubulin and a mitochondrial targeting signal, respectively), which are all correctly co-localized. Each image has a width of 54 μm. (j) Spectral imaging microscopy of single cells expressing a CFP–YFP tandem fusion protein. The data show increased CFP emission and increased sensitized emission (due to FRET) by the mTurquoise2–SYFP2 tandem (n=15) compared with mTurquoise-SYFP2 (n=14). All spectra are normalized to directly excited SYFP2 fluorescence. (k) Photostability of CFP variants was measured in living HeLa cells (n=7, three independent experiments) on wide-field illumination with 436 nm light at an intensity of 1.6 W cm−2, showing that mTurquoise2 is the most photostable CFPin vivo(mTurquoise photostability is identical to mTurquoise2 and has been omitted for clarity). Figure 6: Characterization of the in vivo properties of mTurquoise2. ( a – i ) Fluorescence microscopy images of HeLa cells expressing mTurquoise2 fused to various proteins and targeting sequences (a peroxisomal targeting sequence, Lifeact, no fusion, histone 2A, a nuclear export sequence, a palmitoylation sequence, an endoplasmic reticulum targeting sequence, alpha-tubulin and a mitochondrial targeting signal, respectively), which are all correctly co-localized. Each image has a width of 54 μm. ( j ) Spectral imaging microscopy of single cells expressing a CFP–YFP tandem fusion protein. The data show increased CFP emission and increased sensitized emission (due to FRET) by the mTurquoise2–SYFP2 tandem ( n =15) compared with mTurquoise-SYFP2 ( n =14). All spectra are normalized to directly excited SYFP2 fluorescence. ( k ) Photostability of CFP variants was measured in living HeLa cells ( n =7, three independent experiments) on wide-field illumination with 436 nm light at an intensity of 1.6 W cm −2 , showing that mTurquoise2 is the most photostable CFP in vivo (mTurquoise photostability is identical to mTurquoise2 and has been omitted for clarity). Full size image We hypothesized that, besides the improvement in QY, the improved maturation of mTurquoise2 as compared with mTurquoise would be beneficial for FRET measurements. Therefore, we directly compared the emission spectra of mTurquoise-SYFP2 and mTurquoise-SYFP2 in living cells on excitation of the donor, normalized to the directly excited acceptor signal [10] . It is clear from Fig. 6j that both the CFP and YFP emission are increased for mTurquoise2–SYFP2, demonstrating the increased brightness of mTurquoise2 and the increased sensitized emission from YFP due to enhanced FRET, respectively. In addition, we compared the emission spectra of mTurquoise–SYFP2 and mTurquoise2–SYFP2 in the FRET situation with those of a non-FRET control, again showing the improved brightness of mTurquoise2 in both situations ( Supplementary Fig. S8 ). To examine whether mTurquoise2 is suitable for long-term live-cell imaging, we examined the photostability of mTurquoise2 and compared it with several CFP variants. Initially, we measured photostability with high-intensity excitation light and observed relatively little difference between different CFP variants ( Supplementary Figs S9 and S10 ). However, when the photostability was measured in living cells using lower light intensities that mimic illumination conditions that are typically used for live-cell imaging, we noticed large differences in photostability ( Fig. 6k ). mTurquoise2 and mTurquoise have equal photostability, which is the highest of the CFP variants that were tested ( Table 1 ). Strikingly, mCerulean3, which was reported to have increased photostability in vitro , shows rapid photobleaching in cells. Similar observations were made in different mammalian cell types ( Supplementary Fig. S11 ). From these photobleaching data, we calculated that, at 1.6 W cm −2 illumination conditions, mTurquoise2 emits 1,600,000 photons before photobleaching ( Supplementary Note 2 ; Supplementary Table S5 ), a number that compares favourably with the estimated 400,000 photons emitted by GFP [17] . Reversible photobleaching is of concern for quantitative imaging and has been described for ECFP in vivo [18] , although the effect under physiological conditions is small (<3%) and has not hindered wide application of ECFP as a FRET donor. Although we reproduced the effect for ECFP, we did not observe reversible bleaching in cells expressing mTurquoise2 under the same conditions ( Supplementary Fig. S12 ). All known homologues of GFP found in nature have their chromophore formed from a tyrosine. Proteins with a tryptophan-based chromophore only result from bioengineering initiatives first attempted 18 years ago [2] . As a consequence, CFPs have not benefited from the natural evolution that helped tune the fluorescence quantum yield of tyrosine-based chromophores to high values. For instance, VFP from Cyphastrea microphtalma , plamGFP from Platygira lamellina , sarcGFP from Sarcophyton sp., wild-type GFP from A. victoria , zFP506 from Zoanthus sp. and cFP484 from Clavularia sp. exhibit QYs as high as 1.00, 0.96, 0.96, 0.80, 0.63 and 0.48, respectively [19] , [20] , [21] . Structural reasons for high QY include an environment ensuring the planarity of the chromophore [22] and restriction of its rotational freedom [23] , which primarily occurs through H-bonds between its tyrosyl oxygen and neighbouring residues. In CFPs, stabilization of the chromophore has to occur primarily through an H-bond to the nitrogen atom of the indole ring. Luckily, the original serine at position 205 in A. victoria GFP could serve that purpose. However, it now seems that, during the rational design of ECFP, when extra mutations were required to accommodate the increased bulk of the chromophore, the choice of the S65T mutation was somehow detrimental. This mutation was originally introduced in GFP to favour a deprotonated chromophore, which resulted in the bright cyan-light-excitable EGFP. We show here that the S65T mutation is indeed disadvantageous to the fluorescence properties of CFPs because it modifies the position of Ser205 and weakens its H-bond to the chromophore. Stabilization of the chromophore in mTurquoise occurs by a seemingly modest gain in interaction, which illustrates that the chromophore is already very well stabilized in SCFP3A. However, the key to understand the improvement is that there is a redistribution of interaction energies all around the chromophore. The notably weakened interactions, in particular those with Val150, Ile167 and Ser65 are of vdW nature, which means that they are diffuse. On contradistinction, the most strengthened interactions are localized interactions with Glu222 and Ser205 where the electrostatic forces come into play. Overall, the slight vdW interaction destabilization is more than compensated by the electrostatic interaction stabilization, which contributes to a better positioned chromophore in the excited state. In a previous study, we proposed that the structural modification of the seventh strand of the β-barrel between tyrosine-based and tryptophan-based fluorescent proteins from A. victoria was due to the mutation of a hydrophilic into a hydrophobic amino-acid side chain in the middle of the strand [7] . Indeed, the hydrophobic character of the side chain at position 146 is retained in mTurquoise2. Moreover, the extended size of the side chain allows it to approach closer to the chromophore and establish a set of vdW interactions that is much more extensive than in mTurquoise and previous mutants. As a result, the seventh strand, which is seen to be dynamic in those mutants, is locked into place and the chromophore is now stabilized from all sides. The enhancement of interactions in the chromophore-binding pocket is the explanation for the fluorescence quantum yield close to unity. It is worth mentioning that the various gains in stabilization energy of the chromophore observed in this study do not affect its π electron system, unlike in YFP [24] and mCerulean2.N [12] , where the key mutation occurs at a position orthogonally close to the delocalized electron cloud of the chromophore, lowering the energy of the excited state of the chromophore, thus inducing a redshift in the absorption and fluorescence emission spectra. In contrast, electronic energy levels of the CFP chromophore are unaffected in all the mutants studied here, where mutations occur at positions lateral to the chromophore. Through a combination of structure-guided rational design and fluorescence lifetime screening, we were able to obtain a monomeric fluorescent protein with the highest quantum yield to date (QY=0.93). Moreover, mTurquoise2 shows improved performance in vivo due to better maturation that contributes to an increase of its brightness in mammalian cells of almost 20%. Because of its high quantum yield, mono-exponential fluorescence lifetime, improved maturation rate, and high photostability in vivo , mTurquoise2 is the preferable CFP variant for live-cell imaging and FRET studies with a YFP. We believe that opportunities for furthere improvements in brightness and excited state lifetime may now have been exhausted in this spectral class of A . victoria -derived fluorescent proteins. We have developed an integrated strategy combining structural analysis, site-directed random mutagenesis, and high-throughput screening by FLIM to increase the fluorescence quantum yield of a fluorescent protein close to unity. Such an approach is very likely to be applicable to the wealth of tyrosine-based fluorescent proteins for which there is still room for substantial improvements. Protein expression and purification The K206A mutation was introduced by mutagenesis in SCFP3A, mTurquoise and mTurquoise2 on the pRSET vector (primers listed in Supplementary Table S6 ). After verification by sequencing, the coding sequence of the CFP variants was transferred into pQE60–Cerulean [7] , using the Nco I and Bsr GI restriction sites to replace Cerulean. His-tagged recombinant proteins meant for crystallization were expressed in E. coli BL21 CodonPlus (DE3) RIL cells (Stratagene) in autoinduction medium, at 27 °C for 24 h on the RoBioMol platform of the Institut de Biologie Structurale. Cells were lysed by sonication in the presence of 20 mM Tris (pH 8.0) and 500 mM NaCl with EDTA-free protease inhibitors (Complete, Roche). His-tagged proteins were purified on a Ni-NTA Superflow column (Qiagen) and eluted with 100 mM imidazole in the buffer described above. Fractions containing purified proteins were pooled, dialysed against 20 mM Tris (pH 8.0), and concentrated to 38–85 mg ml −1 . Site-directed mutagenesis of pRSET-mTurquoise on position 146, 165 or 220 were performed using the primers listed in Supplementary Table S6 . For spectroscopic characterization, proteins were expressed using the pRSET vectors expressed in BL21 (DE3) cells and purified as described [10] . Spectroscopic characterization of purified protein Ultraviolet-visible light absorption was measured on a Libra double-beam spectrophotometer (Biochrom). Extinction coefficients were determined from purified protein samples by measuring the absorbance and determining the amount of protein via the BCA assay (Pierce). Quantum yields of protein diluted in PBS buffer (OD 455 <0.05) were determined by excitation at 455 nm (slit 1 nm) and emission measured from 460–650 nm (slit 2 nm) on a PTI QuantaMaster 2000-4 fluorescence spectrofluorometer (Photon Technology International) and subsequent comparison of the integrated fluorescence to the standard fluorescein (QY=0.92 in 0.1 M sodium borate pH 9.1) as described [25] . In vitro brightness Samples were prepared by lysing transfected HeLa cells in PBS containing 1% Triton X-100 and subsequent dilution into PBS with 0.01%. Triton X-100, or by diluting purified protein in 20 mM Tris or PBS with 0.01% Triton X-100, all with the same results. Fluorescence fluctuation spectroscopy was performed on an inverted Fluoview 1000 laser scanning microscope (Olympus). The excitation light of a 440-nm 20-MHz pulsing laser diode (Picoquant), as controlled by a SepiaII laser driver unit (Picoquant), was attenuated 10 times by a neutral density filter. The light was guided via a D440/514/594 primary dichroic mirror (Chroma Technology) through a water immersed ×60 UPlanSApo objective (NA 1.2) into the sample. The emission light was guided via a size-adjustable pinhole, set at 120 μm, through the Olympus detection box to the fibre output channel. The optical fibre was coupled to a custom-made detection box (Picoquant) containing four PDM avalanche photodiodes. The light was guided into one of the PDM avalanche photodiodes where the light was filtered by a 475/45 emission filter (Chroma). The photon arrival times were recorded by a Picoharp 300 time-correlated single-photon counting system (Picoquant) during 120–240 seconds, controlled via the SymPhoTime 5.13 (Picoquant) software. The size and shape of the observation volume was determined from FCS measurements of the calibration dyes Atto425 (AttoTec) as outlined [26] . The molecular brightness of the CFP variants was analysed by photon-counting distribution analysis in FFS Data Processor 2.3 software (SSTC), essentially as described before [10] . The data was binned in time windows of 0.1, 0.5, 1 and 5 ms and analysed using an one-component three-dimensional diffusion model [27] . Crystallization, data collection and structure refinement SCFP3A, mTurquoise and mTurquoise2 all contain the spectroscopically silent A206K mutation known to abolish the weak dimerization that is observed for A. victoria fluorescent proteins at high concentrations [28] . Although we managed to crystallize one of these mutants, we obtained crystals more reliably of the dimeric variants K206A. As the structure of the A206K mutant was virtually indistinguishable from that of the K206A one, apart from the presence of the lysine side chain, we chose the dimerizing versions for structural characterization, and used them as models for the structures of SCFP3A, mTurquoise, and mTurquoise2. Proteins were crystallized using the hanging drop method at 20 °C, at a 13–35 mg ml −1 concentration, in 8–23% PEG8000, 100 mM MgCl 2 , and 100 mM HEPES pH 6.5–7.5. Crystals grew as long thin needles of typically 10–30 μm thickness, well-suited for helical data collections [29] . Data sets were recorded at 100 K at the European synchrotron radiation facility in Grenoble on beamlines ID23-eh1 (wavelength 1.033 Å) for SCFP3A and ID29 (wavelength 0.976 Å) for mTurquoise and mTurquoise2. Data sets were integrated with XDS [30] , then scaled and merged with SCALA [31] . The 1.15 Å structure of Cerulean [7] was used for molecular replacement (PDB ID: 2wso), where all waters, the chromophore and the seventh strand of the protein were removed. Structures were refined with REFMAC with anisotropic temperature factors [32] and model building was performed in COOT [33] . Out of the 221 analysable residues modelled for SCFP3A and mTurquoise, one is an outlier (Asn144) and four are in allowed regions of the Ramanchandran plot, as determined in COOT. Correspondingly, for mTurquoise2, of which the complete sequence of the protein could be modelled, one residue is an outlier (Asn144), and five are in allowed regions, out of 232 analysable residues. Data reduction and structure refinement statistics can be found in Table 2 . Fourier difference maps were calculated using the programs CAD, SCALEIT and FFT from the CCP4 suite [31] . Two different difference maps could be calculated from two sets of SCFP3A and mTurquoise structures and proved to be very similar. The quality of the electron density of the mTurquoise2 structure can be assessed by the stereo view Supplementary Fig. S13 featuring the chromophore and neighbouring residues. Structural alignments based on β-strand C α s were performed in PyMOL ( http://www.pymol.org/ ), excluding those of the seventh strand. Figures of structures were prepared with PyMOL. Table 2 X-ray data collection and refinement statistics. Full size table Spectroscopic characterization of crystals Ultraviolet-visible light absorption spectra, fluorescence emission spectra and TCSPC histograms were recorded of protein crystals and solutions at room temperature or cryocooled at 100 K at the Cryobench facility of the ESRF as previously described [34] . Cryoprotection was assured by addition of 25% glycerol (v/v) to the crystal mother liquor or protein solution. Fluorescence excitation was performed by using 440 nm lasers (CrystaLaser). Interaction energy calculations The proteins SCFP3A, mTurquoise and mTurquoise2 were modelled in solution, using the fDynamo library [35] . The structures of the proteins were first energy-minimized in the ground state (S 0 ) with the optimized potentials for liquid simulations–all-atoms force field [36] . To model the excited state (S 1 ) structures of the proteins, photo-induced changes of electron density on the chromophore were calculated with a hybrid quantum mechanical/molecular mechanical potential [35] ( Supplementary Tables S7 and S8 ). Energies of interactions between residue side chains were calculated by summing the electrostatic and vdW components, in the ground state (S 0 ), and after both instantaneous transition and relaxation in the excited state (S 1 ) ( Supplementary Tables S2 to S4 ). Details of all calculations are provided in Supplementary Note 1 . Fluorescence lifetime imaging Fluorescence lifetime imaging microscopy, multifrequency FLIM and lifetime-based screening were performed, as described [10] . In vivo characterization Expression of mTurquoise and its variants in E. coli was measured at 37 °C using a fluorescence microplate reader, as described [9] , except that we used the pRSET plasmids for expression without induction. For brightness studies in mammalian cells, mTurquoise variants were excised from the pRSET vector using Nhe I and Bsr GI and ligated into the CFP-2A-SYFP2 co-expression vector that was partially digested with Nhe I and BsrG I, and brightness analysis was performed as described [10] 2 days after transfection. For expression of mTurquoise variants in HeLa cells, we replaced the fluorescent protein from pSCFP3A-C1 with the mTurquoise variant using Age I/ Bsr GI restriction sites. Photostability was measured in living HeLa cells by continuous illumination with light from a 100 W mercury lamp that was passed through a 436/20-nm excitation filter and reflected onto the sample with a 455DCLP dichroic mirror (Chroma). A ×63 oil immersion objective (Plan Apochromat NA 1.4) was used and a light intensity of 1.4–1.6 W cm −2 was determined when a ND1.3 grey filter was used, whereas a light intensity of 22–23 W cm −2 was determined without grey filter. To evaluate photostability under laser scanning conditions, we used HeLa cells expressing CFP variants tagged with histone 2A. A Nikon A1 laser scanning microscope was used and cells were imaged using a Nikon Plan Apo VC ×60 oil objective and a zoom factor of 6. Excitation was at 443 nm, and fluorescence was passed through a completely opened pinhole and a 482/35-nm bandpass filter. All parameters, including detector gain, laser intensity, and scan speed were identical between samples. Spectral imaging microscopy was performed on single cells as described [10] . Accession codes: Atomic coordinates and structure factor amplitudes have been deposited in the Protein Data Bank ( http://www.pdb.org/ ) under PDB IDs 2ydz , 2ye0 and 3ztf for SCFP3A, mTurquoise and mTurquoise2, respectively. How to cite this article: Goedhart, J. et al . Structure-guided evolution of cyan fluorescent proteins towards a quantum yield of 93%. Nat. Commun. 3:751 doi: 10.1038/ncomms1738 (2012).